Surface-enhanced redox chemistry of polysulphides on a metallic and polar host for lithium-sulphur batteries The lithium-sulphur battery relies on the reversible conversion between sulphur and Li 2 S and is highly appealing for energy storage owing to its low cost and high energy density. Porous carbons are typically used as sulfur hosts, but they do not adsorb the hydrophilic polysulphide intermediates or adhere well to Li 2 S, resulting in pronounced capacity fading. Here we report a different strategy based on an inherently polar, high surface area metallic oxide cathode host and show that it mitigates polysulphide dissolution by forming an excellent interface with Li 2 S. Complementary physical and electrochemical probes demonstrate strong polysulphide/Li 2 S binding with this ‘sulphiphilic’ host and provide experimental evidence for surface-mediated redox chemistry. In a lithium-sulphur cell, Ti 4 O 7 /S cathodes provide a discharge capacity of 1,070 mAh g −1 at intermediate rates and a doubling in capacity retention with respect to a typical conductive carbon electrode, at practical sulphur mass fractions up to 70 wt%. Stable cycling performance is demonstrated at high rates over 500 cycles. Rechargeable batteries with high energy density and long-lasting cycle performance are highly sought-after for electric vehicles and large-scale electrochemical energy-storage systems. However, current Li-ion batteries using electrodes based on Li + -ion insertion chemistry cannot satisfy this demand in terms of specific energy [1] , [2] . Elemental sulphur—abundant and nontoxic—has become one of the most promising positive electrode active materials because of its high theoretical specific capacity (1,675 mAh g −1 ), based on a redox reaction that reversibly interconverts sulphur and Li 2 S via intermediate lithium polysulphides (LiPSs, that is, Li 2 S n with n =4–8) [3] , [4] , [5] . Li-S cells generally experience low sulphur utilization and poor long-term cycling mainly because of three factors: poor conductivity of sulphur and its discharge products, a large volumetric expansion upon the formation of Li 2 S, and the dissolution of LiPS intermediates in liquid electrolytes, which triggers a polysulphide-shuttle process [3] , [4] , [5] . The latter results in low Coulombic efficiency unless the lithium electrode is passivated. The role of additives in protecting the lithium surface has been thoroughly elucidated [6] , re-inspiring the development of ‘catholyte’-type cells, where the LiPS is completely solubilized. These benefit from tailored cathode architecture designs, such as those based on woven carbon nanotubes [7] . In the opposite tactic where polysulphide dissolution is constrained to increase volumetric energy density, a variety of approaches have been explored. These include solid-state electrolytes [8] , [9] , [10] that show much promise for future development in conjunction with an ionically conductive sulphur cathode [11] . More effort, to date, has been devoted to the cathode side in order to physically confine the LiPSs within the pores or layers of carbonaceous materials that include mesoporous carbon [12] , hollow porous carbon spheres [13] , [14] , graphene [15] , [16] , conductive polymer nanotubes [17] and carbon interlayers [18] . However, over long-term cycling, the hydrophilic LiPSs diffuse out from the hydrophobic pores. This is suspected to be because carbon, being non-polar in nature, does not bind favourably to the polar and ionic sulphides. A more targeted approach is to utilize chemical interactions between oxygen-containing functional groups and the LiPS species on the interface. First employed for polyethylene glycol grafted on mesoporous carbon [12] , more recent studies have demonstrated binding of LiPSs using graphene oxides [19] , [20] or carbon materials decorated with an amphiphilic polymer [21] . However, the functional oxygen-containing groups either lower the overall electronic conductivity or are not permanently bound. Metal oxides, such as SiO 2 (ref. 22 ), TiO 2 (refs 23 , 24 ) and Al 2 O 3 (ref. 25 ) have also been utilized as both adsorbents, and coatings, to hinder the diffusion of LiPSs. Among these, polysulphide reservoirs rely on an insulating mesoporous oxide that traps the LiPS species without directly enabling their reduction [22] , [23] . Nonetheless, insulating oxides ultimately impede electron transport and Li + -ion pathways, thus leading to lower sulphur utilization and rate capability. Seminal work on metal-organic frameworks has shown that these effectively encapsulate LiPSs [26] , and a recent study has elucidated the role of their Lewis acid metal centres in polysulphide adsorption [27] . Although this confirms the importance of chemical interactions in hindering the migration of soluble polysulphides, the intrinsically low electrical conductivity nonetheless results in a relatively low specific discharge capacity of ~650 mAh g −1 . Addressing these limitations is a key point to obtain better electrochemical properties. Here, instead of relying solely on porosity to physically confine sulphides, we present a different approach based on a two-in-one strategy: creation of a bifunctional sulphur host material that combines inherent metallic conductivity with the ability to chemically bind LiPSs on the surface and facilitate reduction to Li 2 S. A high surface area Magnéli phase (Ti 4 O 7 ) fulfills these roles and realizes excellent cycle performance and high-rate capability. While exhibiting bulk metallic conductivity as high as 2 × 10 3 S cm −1 at 298 K [28] , Ti 4 O 7 also contains polar O-Ti-O units that have a high affinity for LiPSs. The presence of strong metal oxide-polysulphide interactions are demonstrated using X-ray photoelectron spectroscopy (XPS), X-ray absorption near-edge structure (XANES) and LiPS adsorption studies. Moreover, by comparison with hydrophobic carbonaceous materials, Li 2 S wetting with the Ti 4 O 7 support is enhanced. This approach to cathode design results in low capacity fade rates for composites containing up to 70 wt% sulphur, even without special binders or surfactants. Material characterization Ti 4 O 7 is a member of the Ti n O 2n−1 Magnéli phases, substoichiometric compositions of metallic titanium oxides that form a homologous series between the end members TiO 2 and Ti 2 O 3 . Their structures are characterized by two-dimensional shear plane slabs of Ti-O octahedra. Ti 4 O 7 has been utilized as a Pt catalyst support for fuel cells because of its high electronic conductivity (about threefold greater than graphite) [29] ; however, its utilization in an ultrahigh surface area modification, which is essential for optimal sulphide interaction, has not yet been reported for energy-storage applications. We synthesized this material by a simple polymer-mediated route (see Methods for details) that relies on the crosslinking of titanium ethoxide with polyethylene glycol followed by carbothermal reduction to crystallize the desired oxygen-deficient titanium oxide. The X-ray diffraction pattern ( Fig. 1a ) indicates that Ti 4 O 7 is the primary crystalline phase; elemental microanalysis indicates the inclusion of 15.4 wt% residual amorphous carbon. The latter is important both to maintain a high surface area and to serve as a hydrophobic component for binding sulphur. High-resolution transmission electron microscopy (TEM) images ( Fig. 1b ) combined with bright/dark field imaging ( Supplementary Fig. 1a,b ) reveal that the material primarily comprises ~8–20 nm Ti 4 O 7 crystals that are loosely bound with interspersed carbon. This gives rise to a bulk four-point probe electronic conductivity on pressed pellet of 3.2±0.1 S cm −1 , which is naturally lower vis a vis the single crystal material but more than sufficient for excellent electron transport within the electrode. The resultant material exhibits a very high surface area of 290 m 2 g −1 (see N 2 adsorption/desorption measurements, Supplementary Fig. 2a ), which is a factor of 100 times higher than conventional Ti 4 O 7 (ref. 30 ). This is essential for interfacial interaction with LiPSs upon cycling as will be demonstrated below. The isotherm measurement also shows the presence of micro and mesopores ( Supplementary Fig. 2b ) that provide both surface area and additional spatial confinement. 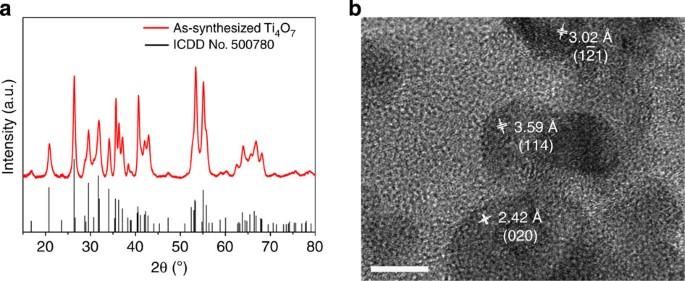Figure 1: Physical characterization of the synthesized Ti4O7. (a) X-ray diffraction pattern and (b) high-resolution TEM image of the Ti4O7nanocrystallites with lattice planes indexed as indicated. Scale bar, 10 nm. Figure 1: Physical characterization of the synthesized Ti 4 O 7 . ( a ) X-ray diffraction pattern and ( b ) high-resolution TEM image of the Ti 4 O 7 nanocrystallites with lattice planes indexed as indicated. Scale bar, 10 nm. Full size image The Ti 4 O 7 was impregnated with 60–70 wt% sulphur by melt-diffusion at 155 °C, determined by thermogravimetric analysis ( Supplementary Fig. 2c ). In addition to intrusion into the pores, sulphur forms a conformal coating on the reduced oxide, as shown using scanning electron microscopy (SEM, Supplementary Fig. 1c ). Energy-dispersive X-ray elemental mapping confirmed a uniform distribution of sulphur over the Magnéli oxide surface ( Supplementary Fig. 3 ). To demonstrate the advantages of conductive oxide materials as a sulphur host versus carbonaceous materials, VULCAN XC72 carbon (denoted as VC) with a similar surface area of 260 m 2 g −1 was used as a comparison. The interaction between Ti 4 O 7 and polysulphides The interaction of different sulphur host materials (Ti 4 O 7 , VC and graphite) with LiPSs was probed using a combination of XPS and visual discrimination, taking Li 2 S 4 as the representative polysulphide. The latter was prepared using previously reported methods [31] . An equivalent amount of target host material (based on surface area) was first added to a solution of Li 2 S 4 in tetrahydrofuran. The superior intrinsic capability of Ti 4 O 7 to adsorb Li 2 S 4 was clearly obvious, as shown in Fig. 2b,c . Addition of Ti 4 O 7 rendered the Li 2 S 4 solution light yellow immediately upon contact and almost completely colourless after it was stirred for 1 h—indicating strong adsorption—whereas the graphite or VC solutions remained intense yellow-gold, indicative of no interaction. 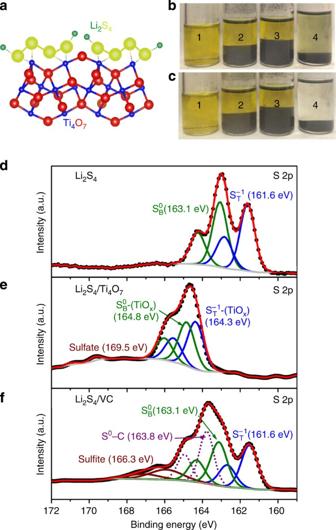Figure 2: Demonstration of the strong interaction of LiPS with Ti4O7. (a) A schematic showing the electron density transfer between Li2S4and TiOx(yellow=S, green=Li, blue=Ti, red=O). (b,c) Sealed vials of a Li2S4/THF solution (1), and after contact with graphite (2), VC carbon (3) and Ti4O7(4), immediately upon contact (b) and after 1 h stirring (c). (d–f) High-resolution XPS S 2pspectra of (d) Li2S4, (e) Li2S4/Ti4O7and (f) Li2S4/VC (black dotted line=experimental data, red line=overall fitted data, solid/dotted lines in other colours=fitted individual components). Figure 2: Demonstration of the strong interaction of LiPS with Ti 4 O 7 . ( a ) A schematic showing the electron density transfer between Li 2 S 4 and TiO x (yellow=S, green=Li, blue=Ti, red=O). ( b , c ) Sealed vials of a Li 2 S 4 /THF solution (1), and after contact with graphite (2), VC carbon (3) and Ti 4 O 7 (4), immediately upon contact ( b ) and after 1 h stirring ( c ). ( d – f ) High-resolution XPS S 2 p spectra of ( d ) Li 2 S 4 , ( e ) Li 2 S 4 /Ti 4 O 7 and ( f ) Li 2 S 4 /VC (black dotted line=experimental data, red line=overall fitted data, solid/dotted lines in other colours=fitted individual components). Full size image The spectrum of Li2S4 materials were analysed using XPS after centrifugation and drying and the S 2p spectra are shown in Fig. 2d–f . Only the 2p 3/2 component of the 2p 3/2 /2p 1/2 doublet is quoted, following convention. The spectrum of Li 2 S 4 ( Fig. 2d ) shows a 1:1 ratio of two 2p3/2 contributions at 161.6 and 163.1 eV, as expected for the terminal () and bridging sulphur (), respectively ( Supplementary Table 1 ). The assignment is based on comparison with values reported for copper polysulphides [32] and the similarity of the spectrum to that of other polysulphides we synthesized ( Supplementary Fig. 4a,b ). The assignment is in accord with the proposed chain-like structure of LiPSs where ab initio calculations show that the negative charge is localized at the termini. [33] The spectrum of Li 2 S 4 bound to Ti 4 O 7 is very different: it exhibits two higher binding energy contributions at 164.3 and 164.8 eV ( Fig. 2e ), representing a +2.7 and +1.7 eV shift for and , respectively. A similar binding energy (164.3 eV) has been attributed to interaction of elemental sulphur with oxygen groups [33] . Although the precise nature of the binding of the sulphide with the metallic oxide is not yet elucidated, data clearly indicate that interaction of both the terminal and bridging sulphur in the LiPS with Ti 4 O 7 surface results in the polarization of electrons away from the sulphur atoms to the electropositive titanium and/or oxygen vacancies at the interface ( Fig. 2a ). The terminal sulphur is more affected owing to its higher electron density. A relatively small shift of −0.2 eV to lower binding energy in the Ti 2p spectrum was also observed indicating increased electron density at the metal centre ( Supplementary Fig. 4d,f ). A chemical reaction such as oxidation of Li 2 S 4 by the Ti 4 O 7 host can be ruled out as a source of the shift, since the oxide has a lower redox potential (~1.75 V; typical of that of slightly reduced titanium oxides) [34] . This is confirmed by the fact that the discharge profile and voltage of the Li 2 S 4 /Ti 4 O 7 is very different than elemental sulphur ( Supplementary Fig. 5 ). We further note that binding energy shifts of a similar magnitude (1.1–3.8 eV) have been predicted on the basis of theory, and experimentally recorded, for anions such as NO x n− species adsorbed on alumina clusters [35] . The minor, broad background contribution between 166 and 169.5 eV on S 2p spectra ( Fig. 2e,f ) is characteristic of sulphite or sulphate [36] arising from a trace amount of water in the solvent. In contrast, the S 2p spectrum of Li 2 S 4 /VC shows two contributions at 161.6 and 163.1 eV, identical to that of Li 2 S 4 ( Fig. 2f ). This, along with the intense colour of the Li 2 S 4 solution even after long-term contact with VC, suggests that almost no adsorption occurs, resulting in essentially unaltered Li 2 S 4 spectral features. An additional peak at 163.8 eV ( Fig. 2f ) is at the same energy for elemental sulphur supported on carbon (S 0 -C) [37] . Similar results were obtained for Li 2 S 4 /graphite ( Supplementary Fig. 4c ). This can be explained by the fact that where little or no interaction of LiPSs with support is present—as in the case of VC and graphite—the polysulphide species exist in rapid equilibria in solution. Disproportionation of intermediate-length LiPSs such as S 4 2− to sulphur with lower and higher oxidation states is known to occur under these conditions [38] , [39] . Shifting of the equilibrium towards elemental sulphur formation is driven both by its insolubility and strong interaction with the carbon surface, thus accounting for the C-S 0 contribution. The accompanying (lower oxidation state) LiPS does not contribute significantly to the averaged spectrum (that is, of the ‘Li 2 S 4-x ’) as long as the extent of the disproportionation reaction remains minor. These findings are in full accord with the LiPS adsorption studies described above. The electrochemical performance of Ti 4 O 7 /S cathodes To evaluate their electrochemical properties, the Ti 4 O 7 /S composites with either 60 or 70 wt% sulphur were cycled from 1.8 to 3.0 V versus Li/Li + . These performed almost identically. The galvanostatic profiles of the Ti 4 O 7 /S nanocomposite at different current densities (after an initial activation cycle at C/20, Fig. 3a ) exhibit two typical well-defined plateaus at ~2.3 and 2.1 V. There is little increase in polarization with increasing rate, indicating favourable kinetics owing to the high electronic conductivity of the Ti 4 O 7 support and good electrolyte accessibility of the discharged/charged products. The Ti 4 O 7 host itself does not contribute to the capacity of the electrode as it accounts for a capacity of only ~6 mAh g −1 ( Supplementary Fig. 6a,b ). Improved long-term cycling performance compared with Vulcan carbon is very evident ( Fig. 3b ). The Ti 4 O 7 /S-60 cell experienced good capacity retention over 250 cycles at C/2 with a fade rate as low as 0.08% per cycle, whereas the VC/S-60 cell faded at twice the rate, 0.16%. As noted above, the Ti 4 O 7 -S/70 cell exhibited the same performance as that of Ti 4 O 7 -S/60, with 88% capacity retention over 100 cycles at C/2 ( Fig. 3c ). At a rate of C/5, an initial capacity of 1,069 mAh g −1 was achieved with the same capacity retention. 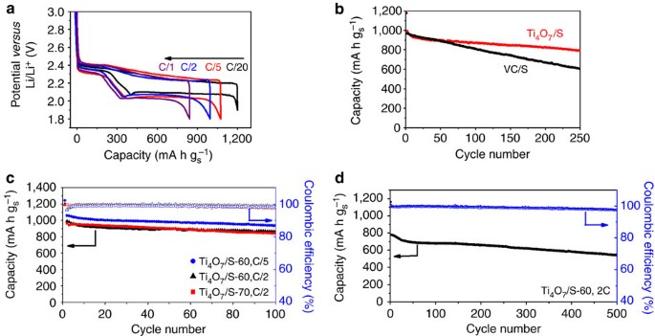Figure 3: Electrochemical performance of Ti4O7/S and VC/S electrodes. (a) Voltage profiles of Ti4O7/S-60-positive electrodes at various rates. (b) Cycling performance of Ti4O7/S-60 and VC/S-60 at C/2 over 250 cycles. (c) Cycling performance of Ti4O7/S composites with different sulphur fractions at C/5 or C/2 over 100 cycles with corresponding Coulombic efficiency. (d) High-rate cycle performance of Ti4O7/S-60 at 2C over 500 cycles with corresponding Coulombic efficiency. The first cycle in all cases was run at C/20 corresponding to an activation cycle (see text). Figure 3d shows high-rate cycling, where an initial capacity of 850 mAh g −1 at 2C was attained for Ti 4 O 7 , with a fade rate of only 0.06% per cycle over 500 cycles. The sulphur/electrolyte ratio was maintained at ~1:30 (g ml −1 ) for both Ti 4 O 7 /S and VC/S cells. To probe the effectiveness of the chemical interaction on the suppression of the polysulphide shuttle, cells without LiNO 3 additive in the electrolyte were also examined. A greatly improved average Coulombic efficiency (~96% versus 80% for VC/S-60) for Ti 4 O 7 /S-60 composite ( Supplementary Fig. 6c,d ) was observed, demonstrating the defining role of the interfacial interaction. Figure 3: Electrochemical performance of Ti 4 O 7 /S and VC/S electrodes. ( a ) Voltage profiles of Ti 4 O 7 /S-60-positive electrodes at various rates. ( b ) Cycling performance of Ti 4 O 7 /S-60 and VC/S-60 at C/2 over 250 cycles. ( c ) Cycling performance of Ti 4 O 7 /S composites with different sulphur fractions at C/5 or C/2 over 100 cycles with corresponding Coulombic efficiency. ( d ) High-rate cycle performance of Ti 4 O 7 /S-60 at 2C over 500 cycles with corresponding Coulombic efficiency. The first cycle in all cases was run at C/20 corresponding to an activation cycle (see text). Full size image Operando XANES study on the Ti 4 O 7 /S electrode Surface-mediated reduction of the sulphide species on Ti 4 O 7 was further confirmed by an operando XANES study. This powerful tool has been previously used by us for monitoring sulphur speciation in Li-S cells [31] , and a significant theoretical understanding of the spectroscopic signatures has been recently reported [40] . Sulphur K-edge spectra collected throughout discharge and charge of a Ti 4 O 7 /S electrode were fitted with a linear combination of α-S 8 , Li 2 S 6 , Li 2 S 4 and Li 2 S and compared with a VC/S electrode. In order to necessarily avoid self-absorption in the XANES experiments [31] and also to preferentially probe the sulphur host interface, both working electrodes were prepared with a low sulphur weight fraction (see details in Supplementary Fig. 7 ). The contributions of the species at various states of discharge are shown in Fig. 4 , with Li 2 S 6 and Li 2 S 4 summed as LiPS for clarity. Compared with a hydrophobic carbon host, the fraction of LiPS intermediates is significantly lessened at all states of discharge (reaching a max of 40% for Ti 4 O 7 versus 87% for carbon, respectively), and Li 2 S precipitates much earlier and more progressively for Ti 4 O 7 . LiPSs chemically adsorbed on the Ti 4 O 7 host are much more readily reduced to Li 2 S than in the case of carbon, as indicated by the reduced overpotential ( Supplementary Fig. 7 ), strongly supporting a more efficient electron transfer from the oxide host to the electroactive mass owing to hydrophilic interactions [19] , [21] , and intimate contact, which leads to increased capacity and longevity. 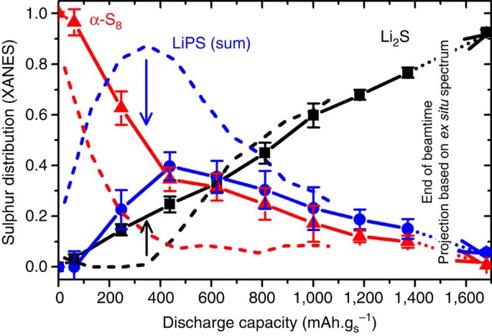Figure 4: Distribution of sulphur species upon discharge determined byoperandoXANES. Data for Ti4O7/S-6 (solid lines+symbols) compared with VC/S-6 (dashed lines) show the much lower concentration of LiPS in solution. Black=Li2S; blue=LiPS, shown as the sum of Li2S6and Li2S4; red=elemental sulphur. SeeSupplementary Fig. 7for experimental spectra and procedures. Figure 4: Distribution of sulphur species upon discharge determined by operando XANES. Data for Ti 4 O 7 /S-6 (solid lines+symbols) compared with VC/S-6 (dashed lines) show the much lower concentration of LiPS in solution. Black=Li 2 S; blue=LiPS, shown as the sum of Li 2 S 6 and Li 2 S 4 ; red=elemental sulphur. See Supplementary Fig. 7 for experimental spectra and procedures. Full size image Morphology of positive electrodes after cycling The underlying reason for the stable capacity delivery was further explored by examining the positive electrode nanostructure evolution over cycling. Cycled cells stopped at different discharged/charged points were disassembled and examined by SEM. 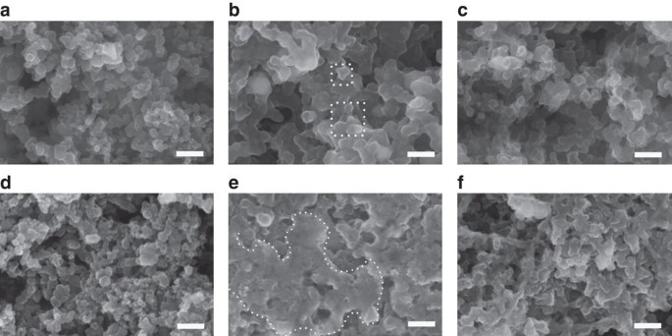Figure 5: SEM images of the Ti4O7/S and VC/S electrodes showing changes with cycling. Images correspond to (a,d) the pristine-positive electrodes and electrodes after (b,e) first discharge where dotted boxes and shapes delineate the Li2S on the support, and (c,f) 500 cycles at charged status for (a–c) Ti4O7/S-60 and (d–f) VC/S-60. Scale bar, 200 nm. Figure 5a,d shows the images for the pristine Ti 4 O 7 /S-60 and VC/S-60 electrodes, respectively. On the first discharge, although an expanded layer of Li 2 S is evident on the surface in both cases, the underlying support is more defined for the Ti 4 O 7 host ( Fig. 5b,e ), indicative of the conformal deposition of Li 2 S on the particle surface as highlighted by the white boxes (the result of better wetting). In contrast, the Li 2 S on carbon is broadly and non-specifically distributed (area encompassed by the dotted white line). This is in agreement with the XANES results that show the gradual deposition of Li 2 S on Ti 4 O 7 (compared with its much more sudden precipitation on carbon, Fig. 4 ). Figure 5: SEM images of the Ti 4 O 7 /S and VC/S electrodes showing changes with cycling. Images correspond to ( a , d ) the pristine-positive electrodes and electrodes after ( b , e ) first discharge where dotted boxes and shapes delineate the Li 2 S on the support, and ( c , f ) 500 cycles at charged status for ( a – c ) Ti 4 O 7 /S-60 and ( d – f ) VC/S-60. Scale bar, 200 nm. Full size image The function of a metallic oxide as a sulphur host is quite different from an insulating oxide such as TiO 2 used as a coating to physically inhibit LiPS diffusion. It also stands in contrast to mesoporous TiO 2 , which functions as a polysulphide reservoir to bind LiPS [22] , or metal-organic frameworks that rely on porosity and acid–base interactions between the LiPS and the metal centre to constrain diffusion. In such oxides, LiPSs cannot engage in redox behaviour at the interface owing to their insulating nature. The metallic oxide, in contrast, triggers surface-mediated reduction of sulphur/oxidation of Li 2 S. This is illustrated in Fig. 6 . On a typical carbon support ( Fig. 6a ), elemental sulphur undergoes reduction to form LiPSs that then dissolve into the electrolyte (as evident in Fig. 2b ). Initial reduction is thought to give S 8 2− that disproportionates in solution to elemental sulphur and S 6 2− (refs 31 , 38 , 39 ). The soluble S 6 2− can either undergo cleavage to form soluble, reducible S 3 − ; or further reduce to S 4 2− and ultimately precipitate Li 2 S; and/or reduce and disproportionate to form a higher order polysulphide and Li 2 S. These solution-mediated reactions are highly complex [38] , [39] . Nonetheless, data clearly show the high concentration or supersaturation of LiPS before the end of discharge ( Fig. 4 ) that results in a broadly distributed deposition of Li 2 S with high interfacial impedance ( Fig. 5e ; Supplementary Fig. 8b ). In the presence of a strong support interaction as witnessed for Ti 4 O 7 , however, our collective results show these processes are significantly affected ( Fig. 6b ). Not only is the concentration of LiPS in solution greatly diminished on discharge but also a slow, controlled deposition of Li 2 S is observed ( Fig. 4 ). This is evidenced not only using XANES but also using the XPS, SEM and impedance data (see below). We ascribe this to the interface-mediated, spatially controlled reduction of the LiPS, where SEM suggests that a conformal coating is produced. 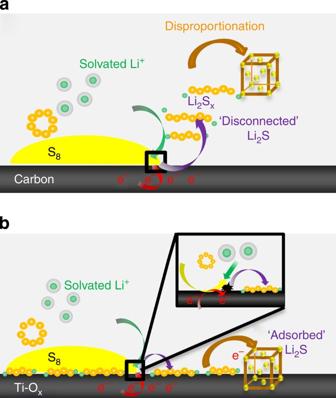Figure 6: Diagram illustrating surface-mediated reduction of Li2S from LiPSs on Ti4O7. (a) On reduction of S8on a carbon host, LiPSs (Li2SX) desorb from the surface and undergo solution-mediated reactions leading to broadly distributed precipitation of Li2S. (b) On reduction of S8on the metallic polar Ti4O7, LiPSs adsorb on the surface and are reduced to Li2S via surface-mediated reduction at the interface. Figure 6: Diagram illustrating surface-mediated reduction of Li 2 S from LiPSs on Ti 4 O 7 . ( a ) On reduction of S 8 on a carbon host, LiPSs (Li 2 S X ) desorb from the surface and undergo solution-mediated reactions leading to broadly distributed precipitation of Li 2 S. ( b ) On reduction of S 8 on the metallic polar Ti 4 O 7 , LiPSs adsorb on the surface and are reduced to Li 2 S via surface-mediated reduction at the interface. Full size image Electrochemical impedance (EIS) spectroscopy on the cycled electrodes lends additional support to the concept of surface-mediated reduction of sulphur ( Supplementary Table 2 ). These studies provide measure of the charge-transfer resistance at the positive (or negative) electrode interface resulting from deposition of products on discharge and charge [41] . On the first discharge, the Ti 4 O 7 /S-60 cell exhibits a charge-transfer resistance in the high-intermediate frequency range (attributable to the positive electrode) that is twofold lower that of the VC/S-60 ( Supplementary Figs 8a,b and 9 ). We ascribe this to the enhanced interaction of the LiPSs—and subsequently the Li 2 S—with Ti 4 O 7 , in full concert with the findings from SEM and XANES data. Thus, as expected, the nonspecific precipitation of Li 2 S on the carbon-based electrode gives rise to higher resistance, whereas charge transfer at the ionic Li 2 S–Ti 4 O 7 interface is more efficient. After the fifth charge or discharge, the Ti 4 O 7 /S-60-positive electrode also exhibited a very similar morphology to the pristine electrode, that is, sulphur (on charge) or Li 2 S (on discharge) was re-deposited on the Ti 4 O 7 support uniformly ( Supplementary Fig. 10a,b ). In accord, EIS spectra at both discharge and charge for Ti 4 O 7 /S-60 over 50 cycles show negligible change ( Supplementary Fig. 8c,d ). Even after 500 cycles at C/2, SEM images of the cathodes show that the original morphology of the electrode structure is better preserved on charge for Ti 4 O 7 /S-60 ( Fig. 5c ) than in the VC/S-60-positive electrode ( Fig. 5f ). In the latter case, this could arise from residual unoxidized Li 2 S, as it has been shown that Li 2 S particles easily detach from carbon electrode surfaces leading to loss in electrical contact [21] . Conversely, for Ti 4 O 7 /S, the maintenance of nanostructure integrity along with the minimal variation in the charge-transfer resistance on cycling demonstrate strong interaction between the host and the (poly)sulphide species. Our results suggest that this allows for their reversible, homogeneous deposition to Li 2 S (and its subsequent oxidation) and accounts for the observed enhanced cell longevity. Cell charging to form elemental sulphur is also assisted by the presence of hydrophobic carbon in the composite. In summary, we have demonstrated a new class of inorganic sulphur host materials that combine electronic conductivity for redox electron transfer with a polar surface for strong LiPSs/Li 2 S binding, which provide a bifunctional positive electrode material for Li-S batteries that enables low capacity fade rates to be sustained. At sulphur fractions comparable to those of mesoporous carbons, electrodes show better cycling stability. This indicates that surface interactions play a larger role in containing sulphide dissolution and deposition than mesoporous confinement that relies on physical barriers. Particularly important in directing gradual reduction to Li 2 S, and enhancing redox electron transfer, this is even more important for lithium sulphide than for sulphur (which is partly soluble), to reduce interfacial impedance. When the sulphur/sulphide host is both sulphiphilic and metallic, redox is further facilitated. The concept extends not only to the other members of the Magnéli phase family but is also widely applicable to conductive materials with intrinsic polar character, as we will show in subsequent reports. This opens the path to a departure from traditional cathode design for Li-S cells based on functionalized carbons and should inspire further studies on the nature of the sulphide–support interaction. These will be particularly important for catholyte cells that will benefit from spatially controlled precipitation of sulphides and lowered charge potentials on charge. Synthesis of Ti 4 O 7 and related sulphur composites In a typical synthesis, titanium(IV) ethoxide (Sigma-Aldrich) and polyethylene glycol (Mw~400, Sigma-Aldrich) were mixed in the desired weight ratio followed by addition of ethanol to control the viscosity. The solution was then stirred at 60–80 °C for overnight to form an amber yellow gel. This gel was further heated at 100 °C for 4–6 h and then fired at ~950 °C under an Ar stream in a tubular furnace using a heating ramp of 4 °C min −1 . A black powder product was obtained. Ti 4 O 7 /S-60 (and Ti 4 O 7 /S-70) were prepared with either 60 or 70 wt% percent sulphur, respectively, via a well-established melt-diffusion method at 155 °C. For comparison, the VC/S-60 composite was similarly prepared from VULCAN XC72 carbon (Cabot Corporation, denoted as VC) with a surface area of 260 m 2 g −1 . Synthesis of lithium and sodium polysulphides for XPS Solid Li 2 S 4 was synthesized by reacting elemental sulphur and lithium superhydride (LiEt 3 BH) in the desired ratio in anhydrous THF at room temperature for 1 h inside an Ar-filled glovebox. The THF was removed in vacuo and the precipitate was washed with toluene and vacuum dried, as reported previously [31] . Na 2 S 2 and Na 2 S 4 as reference materials for XPS were prepared by reacting sodium sulphide nonahydrate with elemental sulphur in the desired ratios in absolute ethanol under an N 2 flow. The mixture was refluxed for 1 h and then cooled down at room temperature for overnight. The powder was dried in vacuo and further heated at 80 °C for 2 h. Polysulphide adsorption study and XPS sample preparation Three Li 2 S 4 solutions were prepared by dissolving 4 mg of Li 2 S 4 in 5 ml of THF in each case. Graphite (Alfa Aesar), VULCAN XC72 carbon (Cabot Corporation) and mesoporous Ti 4 O 7 were added to each solution. The mass added was adjusted so the total surface areas of the solids based on Brunauer–Emmett–Teller measurements were the same (5.8 m 2 ) for each. For example, for Ti 4 O 7 with a surface area of 290 m 2 g −1 , 20 mg were added. To inspect the solution colour, in the first step, immediately upon stirring, the suspensions were allowed to settle for a few minutes. For the second step, the solutions were further stirred for 1 h. Afterwards, the suspensions were centrifuged and the solids for XPS analysis were obtained after drying in vacuo for 5 h. All procedures were completed in an Ar-filled glovebox. Electrochemical measurements Sulphur composites (Ti 4 O 7 /S or VC/S) with Super P and Kynar Powerflex binder at a weight ratio of 8:1:1 were dispersed in dimethylformamide to form a thin slurry that was drop-cast on carbon paper with an area of 2 cm 2 (AvCarb P50, Fuel Cell Store) to prepare the positive electrodes. The electrodes were dried at 60 °C overnight before use. Coin cells were assembled inside the glovebox with lithium foil as anode and an electrolyte consisting of 1 M bis(trifluoromethanesulfonyl)imide lithium and 2 wt% of LiNO 3 in a mixed solvent of 1,2-dimethoxyethane and 1,3-dioxolane (v/v=1:1; BASF). The typical sulphur loading was 1.5–1.8 mg per electrode, with an electrolyte volume of 50 μl in all cases. The cells were galvanostatically cycled between 1.8 and 3.0 V at different C rates (1C=1,675 mA g −1 ) using a BT2000 battery cycler (Arbin Instruments). A voltage window of 1.9–3.0 V was used for cycling at C/20 and 1.7–3.0 V for 2C. EIS measurements were carried out on a VMP3 potentiostat/galvanostat station with EIS/Z capabilities (Bio-Logic Science Instruments). The DC voltage was kept at open-circuit voltage and an AC voltage of 5 mV in amplitude was applied with a frequency of 200 kHz–20 mHz. XANES studies XANES measurements were carried out at the sector 13-ID-E at the Argonne National Laboratory using a Si(111) crystal monochromator under helium flow and the data were collected in fluorescence mode using a four-element vortex detector. The cell used to perform operando XANES was adapted from the 2,325 coin cell as described in ref. 31 . In order to both avoid self-absorption and preferentially probe the sulphur host interface, the working electrodes were made of Ti 4 O 7 /S-6 wt% or VC/S-6 wt%, Super P carbon and polyvinylidene difluoride (1.6 wt% sulphur overall) and were cycled against a LiNO 3 -protected Li-negative electrode in 1 M LiClO 4 , DME:DOL (1:1) electrolyte at a rate of C/5. The experimental spectra acquired operando were compared with a set of reference materials including α-S 8 , Li 2 S 6 , Li 2 S 4 and Li 2 S [31] . Since the standards represent the sulphur species successively formed by electrochemistry, operando spectra can be described with a linear combination fitting [31] , as shown in Fig. 4 and Supplementary Fig. 7 . Preparation of cycled electrode samples for SEM imaging Positive electrodes (Ti 4 O 7 /S-60 and VC/S-60) were retrieved after a specified number of cycles at either a charged or discharged status by dissembling the cells in the glovebox. Electrodes were washed with acetonitrile twice to remove dissolved lithium polysulphides and lithium salt on the surface, followed by drying in vacuo for 30 min. Dried electrodes were then transferred to the SEM chamber under an Ar atmosphere for imaging. Material characterization Elemental microanalysis on the as-synthesized Ti 4 O 7 material was conducted on a Carlo Erba elemental analyzer (CHNS-O EA1108, Italy) coupled to a Delta plus continuous flow stable isotope ratio mass spectrometer (Thermo Finnigan, Bremen, Germany). The X-ray diffraction pattern was collected on a Bruker D8-Advance powder X-ray diffractometer, operating at 40 kV/30 mA and using Cu-Kα radiation ( λ =0.15405, nm). The SEM imaging and EDX elemental mapping were performed using a LEO 1530 field emission SEM equipped with an EDX attachment (Zeiss). The TEM samples were imaged on JEOL 2010F TEM/STEM operating at 200 KeV. N 2 adsorption/desorption isotherms were obtained using a Quantachrome Autosorb-1 system at 77 K. Surface areas were calculated using the Brunauer–Emmett–Teller method based on a multipoint analysis. Ti 4 O 7 , VC and graphite were degassed at 180 °C before measurement. Thermogravimetric analysis was conducted using a TA Instruments SDT Q600 under a N 2 flow at a heating rate of 10 °C min −1 . Electronic conductivity was measured using a Jandel four-point probe connected to an RM3000 test unit. The Ti 4 O 7 powder was pressed into a pellet and sintered at 800 °C under Ar for 12 h before measurement. Different spots and currents were used to obtain an average conductivity value. XPS analysis was performed on a Thermo ESCALAB 250 instrument configured with a monochromatic Al Kα (1,486.6 eV) for conductive composite materials and non-monochromatic Al Kα (from a twin anode) for non-conductive materials (Na 2 S x , Li 2 S 4 and S 8 ). The air-sensitive samples were transported to the spectrometer under an Ar atmosphere and transferred into the chamber anaerobically. All spectra were fitted with Gaussian–Lorentzian functions and a Shirley-type background using the CasaXPS software. For S 2p spectra, three constraints were used on the fitting for 2p 3/2 and 2p 1/2 doublets: (a) a peak position difference of 1.18 eV between them, (b) a peak area ratio of 2:1 for 2p 3/2 : 2p 1/2 and (c) equal full-width half maximum. For the Ti 2p spectrum, a peak position difference of 5.7 eV was used. The binding energy values were all calibrated using the C 1s peak at 285.0 eV. How to cite this article: Pang, Q. et al. Surface-enhanced redox chemistry of polysulphides on a metallic and polar host for lithium-sulphur batteries. Nat. Commun. 5:4759 doi: 10.1038/ncomms5759 (2014).